Unlocking Bloch-type chirality in ultrathin magnets through uniaxial strain Chiral magnetic domain walls are of great interest because lifting the energetic degeneracy of left- and right-handed spin textures in magnetic domain walls enables fast current-driven domain wall propagation. Although two types of magnetic domain walls are known to exist in magnetic thin films, Bloch- and Néel-walls, up to now the stabilization of homochirality was restricted to Néel-type domain walls. Since the driving mechanism of thin-film magnetic chirality, the interfacial Dzyaloshinskii–Moriya interaction, is thought to vanish in Bloch-type walls, homochiral Bloch walls have remained elusive. Here we use real-space imaging of the spin texture in iron/nickel bilayers on tungsten to show that chiral domain walls of mixed Bloch-type and Néel-type can indeed be stabilized by adding uniaxial strain in the presence of interfacial Dzyaloshinskii–Moriya interaction. Our findings introduce Bloch-type chirality as a new spin texture, which may open up new opportunities to design spin–orbitronics devices. The formation of magnetic domains and domain walls (DWs) results from the interplay between the exchange interaction, the dipolar interaction and magnetic anisotropy. In perpendicularly magnetized thin-film systems, DWs can be classified as two canonical types: in Bloch walls, the spin rotates like a helical spiral around an axis which is parallel or antiparallel to the DW normal, whereas in Néel walls the spin rotates like a cycloidal spiral. A magnetic film is called chiral when the rotational sense of these spirals is the same in all DWs. In non-chiral films, both rotation senses exist in different sections of DWs, with the same probability overall. The conventional textbook view predicts non-chiral Bloch walls as the ground state in magnetic thin films [1] , [2] , [3] . In this picture chirality, that is, one preferred spin rotational sense in DWs, does not emerge because the magnetic energy contributions are all symmetric with respect to the rotation direction between to spins. An asymmetric exchange interaction term, known as the Dzyaloshinskii–Moriya interaction (DMI), can be induced when inversion symmetry is broken in the system [4] , [5] . The inversion symmetry can break in the lattice (bulk DMI) or at surfaces and interfaces (interfacial DMI) of magnetic films [6] , [7] , [8] . The DMI term between two atomic spin S i and S j on neighbouring atomic sites i and j can be written as E DM =− D ij ·( S i × S j ), where D ij is the DMI vector. In the case of interfacial DMI, D ij is restricted to be perpendicular to the position vector r ij = r i − r j (refs 6 , 7 , 8 , 9 ). For this reason, interfacial DMI alone can only stabilize Néel-type chiral spin textures, such as cycloidal spin spirals [10] , [11] , [12] , skyrmions [13] , [14] or chiral Néel walls [15] , [16] , [17] . In Bloch-type spin textures, the cross-product ( S i × S j ) is parallel to the position vector r ij and E DM vanishes, consequently Bloch walls are usually non-chiral. It was recently found that chiral Néel walls in film and multilayer structures enable fast current-driven DW motion and spin texture-dependent DW propagation direction [15] , [18] , [19] , [20] , [21] . A numerical study also predicts that introducing chirality of Bloch walls into magnetic films can extend possibilities to manipulate DW propagation behaviours to new geometries [18] . Developing experimental evidence that allows us to tailor the spin structure of chiral DWs via interfacial DMI [6] , [22] is crucial for engineering methods to control current- or field-driven DW dynamics in film and multilayer structures, since these phenomena hold great potential for information storage and spintronics. In particular, direct observations of DW spin structure under the combined effects of interfacial DMI and in-plane uniaxial anisotropy are still missing. In the following, we demonstrate how the introduction of in-plane uniaxial anisotropy allows us to tailor the DMI-stabilized chiral DW spin textures. We focus on Fe/Ni bilayer grown on W(110) substrates, where the very large spin Hall angle of tungsten [23] is combined with two-fold symmetry at the (110) interface and perpendicular magnetic anisotropy of the magnetic layer [24] , [25] , [26] . Using spin-polarized low-energy electron microscopy (SPLEEM) [27] , [28] , [29] , we observe anisotropic chiral DW spin structures with mixed components of chiral Bloch- and chiral Néel-character. We find that, as a function of the relative orientation of the DWs with respect to the [001] substrate surface direction, the Fe/Ni/W(110) system features chiral Néel walls, mixed chiral walls containing both Néel and Bloch components or non-chiral Bloch walls. The chirality of the Néel wall components is always left-handed, whereas the chirality of the Bloch wall components is either left- or right-handed. Bloch-component handedness as well as the ratio of the Bloch- versus Néel- components depends on the orientation relationship between the DW direction and the substrate lattice. Supported by Monte Carlo simulations, we propose that the origin of anisotropic chirality is the interplay between the DMI, the dipolar interaction and the in-plane uniaxial anisotropy. Our findings experimentally demonstrate the Bloch-type chirality as a new type of chiral spin texture stabilized by interfacial DMI, which may open up new opportunities to design spin–orbitronics devices. Visualizing chiral DWs Within DWs in perpendicularly magnetized systems, spins usually rotate from one domain to another in one of the four basic spin textures, which are Bloch- or Néel walls with left- or right-handed chirality. 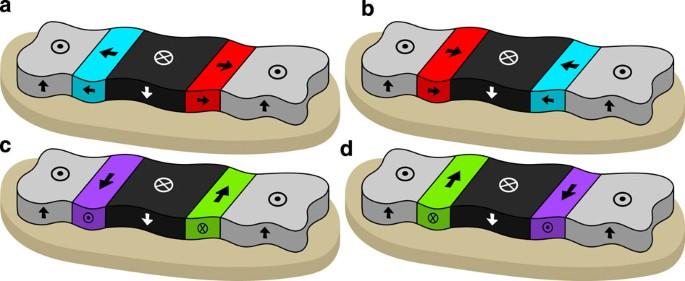Figure 1: Schematic of chiral DWs. Sketch of left-handed (a) and right-handed (b) chiral Néel walls in perpendicularly magnetized thin film, directions of arrows correspond to the magnetization direction. The spin structure of the DW is simplified by highlighting the in-plane component in the centre of the walls. Sketch of left-handed (c) and right-handed (d) chiral Bloch walls in a perpendicularly magnetized thin film. Figure 1 shows sketches of a left-handed (a) and right-handed (b) chiral Néel wall and a left-handed (c) and right-handed (d) chiral Bloch wall. Experimentally, chirality in magnetic DWs can be determined by imaging three-dimensional spin textures. 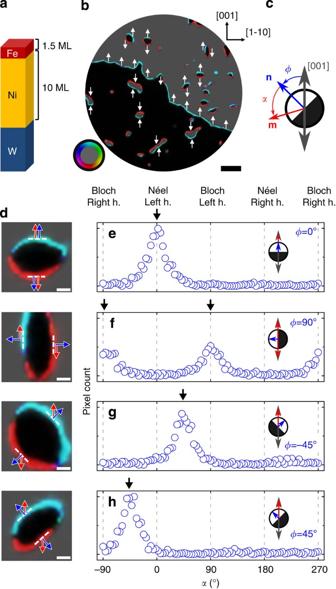Figure 2: Real-space observation of anisotropic chiral DWs in a Fe/Ni bilayer. (a) Profile sketch of Fe/Ni bilayer grown on W(110) substrate. (b) Compound SPLEEM image, colourized DW highlights the in-plane orientation of the magnetization inside the DW; scale bar, 1 μm. (c) Definition of anglesαandφ,mindicates the in-plane component of the DW, blue arrow indicates normal vectorn, grey arrow indicates W[001] direction. (d) Examples of different DW orientations, data are cropped fromb. DW tangent directions are indicated by white dashed lines, scale bars are 100 nm. (e–h)φ-dependent histograms of angleαin DW centre, counted pixel-by-pixel in four SPLEEM compound images includingb. The histograms are normalized with respect to the total number of evaluated states. Left h., left-handed; ML, monolayer; right h., right-handed. Figure 2 shows a SPLEEM measurement of the DW spin structure in a Fe/Ni bilayer grown on W(110) substrate. The structure of the thin film is sketched in Fig. 2a , and a typical compound SPLEEM image (see Methods) is shown in Fig. 2b where blue/yellow indicates magnetization components along [1–10]/[−110] and cyan/red indicates components along [001]/[00-1]. In this rendering scheme, all DWs are highlighted in colour and, in Fig. 2b , we notice that all DWs are either cyan or red, which means that the in-plane components of all DWs are either parallel or antiparallel to W[001], even though the directions of DWs are oriented along all possible directions within the film plane. These findings are reproduced in all images of other areas of this and a number of additional samples (see Supplementary Fig. 1 ). This indicates that the inner spin structure of DWs in the Fe/Ni/W(110) system is coupled to the direction of the DW with respect to the W[001] lattice direction. Figure 1: Schematic of chiral DWs. Sketch of left-handed ( a ) and right-handed ( b ) chiral Néel walls in perpendicularly magnetized thin film, directions of arrows correspond to the magnetization direction. The spin structure of the DW is simplified by highlighting the in-plane component in the centre of the walls. Sketch of left-handed ( c ) and right-handed ( d ) chiral Bloch walls in a perpendicularly magnetized thin film. Full size image Figure 2: Real-space observation of anisotropic chiral DWs in a Fe/Ni bilayer. ( a ) Profile sketch of Fe/Ni bilayer grown on W(110) substrate. ( b ) Compound SPLEEM image, colourized DW highlights the in-plane orientation of the magnetization inside the DW; scale bar, 1 μm. ( c ) Definition of angles α and φ , m indicates the in-plane component of the DW, blue arrow indicates normal vector n , grey arrow indicates W[001] direction. ( d ) Examples of different DW orientations, data are cropped from b . DW tangent directions are indicated by white dashed lines, scale bars are 100 nm. ( e – h ) φ -dependent histograms of angle α in DW centre, counted pixel-by-pixel in four SPLEEM compound images including b . The histograms are normalized with respect to the total number of evaluated states. Left h., left-handed; ML, monolayer; right h., right-handed. Full size image To understand the micromagnetic properties of these DWs, we analyse the spin texture of the DWs in more detail. We start by identifying the image pixels on the centerlines of all DWs in a representative set of SPLEEM images (see Methods). At all centreline-pixels of all the DWs, we measure the local direction of the magnetization, expressed as the magnetization unit vector m , and the direction of the in-plane normal vector n of the DW. We represent these data in terms of two angles: to capture the DW orientation, we define the angle φ as the angle of the normal vector n of the DW with respect to the W[001] lattice direction, and to capture the local DW spin texture, we define the angle α as the angle between the magnetization unit vector m and the in-plane normal vector n of the DW; the geometry of these angles is sketched in Fig. 2c . The magnitude of the angle α indicates whether the wall is in Bloch configuration ( α =±90°) or in Néel-configuration ( α =0° or α =180°) [17] . Our measurements show that not only do both of these DW types occur, but there are also parts of the DWs which exhibit mixed types (for example, α =±45°). We notice that the magnitude of the angle α , and thus the type of the wall, is a function of the orientation of the wall φ. Figure 2d reproduces SPLEEM images cropped from Fig. 2b to show DW sections, highlighted by dashed lines, where certain DW orientations are prevalent (red and blue arrows in the SPLEEM images indicate directions of DW magnetization unit vector m and DW normal vector n within these DW sections). Next to these images, Fig. 2e–h shows histograms of the angle α at DW sections with corresponding orientations. Key points for these data demonstrated are as follows: when DW tangential direction is parallel to [1–10], that is, φ =0°±3°, then the histogram plotted in Fig. 2e shows that the angle α is scattered about a narrow distribution centred near 0°, confirming that these DWs are Néel type with left-handed chirality [17] . When φ =90°±3° (DW tangential direction is parallel to [001], Fig. 2f ), then the distribution of α has two peaks with comparable heights centred at −90° and +90°, indicating right- and left-handed Bloch wall sections. This distribution corresponds to the conventional case of non-chiral Bloch walls [17] . The distribution for φ =−45°±3° is shown in Fig. 2g , where a peak showing a narrow distribution of the angle α appears at ~+45°. Although this is clearly a chiral spin structure, it neither corresponds to chiral Néel wall [15] , [16] , [17] nor to non-chiral Bloch wall [1] , [2] , [3] , [16] , [17] . This DW spin texture can be understood as a superposition of the left-handed chiral Néel structure and left-handed chiral Bloch structure, that is, as in Néel walls the spin vector tilts towards the in-plane normal direction of the DW while, at the same time, it rotates around the DW normal as it does in Bloch walls. We will refer to this texture as a mixed DW. Similarly, when φ =45°±3°, as shown in Fig. 2h , then the single peak at −45° indicates a mixed chiral wall type composed of a left-handed Néel component and a right-handed Bloch-component. Quantitative picture of anisotropic chirality To analyse the orientation-dependent DW structure systematically, we test how Bloch-type chirality evolves from left-handed to non-chiral to right-handed chiral order as seen, for example, in Fig. 2f–h . A two-dimensional histogram reproduced in Fig. 3a shows the statistical likeliness of DW spin configurations α and DW orientations φ ; on our colour scale, rare α / φ combinations are darker and common α / φ combinations are brighter. To guide interpretation, Fig. 3b shows the sketches of DW configurations corresponding to the α − φ histogram plotted in Fig. 3a . As defined in the inset in Fig. 2 , red arrows in Fig. 3b indicate the in-plane direction of magnetization inside the DW and blue arrows correspond to the DW normal n . Vertical cuts along green dashed lines through the two-dimensional histogram in Fig. 3a correspond to the histograms of α as shown in Fig. 2e–h . The bright regions in Fig. 3a (emerald-coloured regions in Fig. 3b ) represent the most common DW spin textures found experimentally. The most prominent feature in this histogram is a diagonal streak in the lower half. This streak forms for two reasons. First, in this region of the histogram, the orientations of in-plane components of DW magnetization (red arrows) are aligned with in-plane uniaxial magnetic anisotropy K u , that is, parallel to the W[001] direction. Second, the Néel components of spin textures in the lower half of the histogram (−90°< α <90°) are always left handed. By contrast, a similar diagonal steak is suppressed in the upper half of the histogram (90°< α <270°) because, although a corresponding region exists where DW magnetization is aligned with K u , the Néel components of spin textures in this part of the histogram are right-handed and thus energetically unfavourable as a result of the DMI of this system. Besides the prominent diagonal steak, six additional DW textures are observed where both α and φ are right angles (four bright regions in the four corners of the histogram and two bright regions where α =90° and φ =±90°). These α / φ combinations correspond to pure Bloch textures. The fact that for φ =−90° and +90° we simultaneously observe textures with α =90° (left-handed) and with α =−90° or α =270° (right-handed) indicates that the system is achiral in the limit of pure Bloch texture. 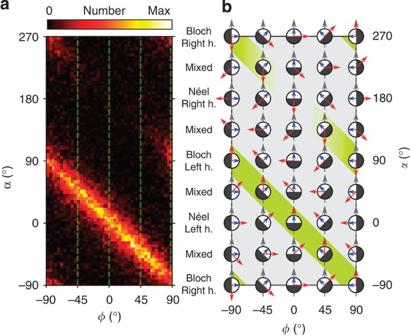Figure 3: Distribution of anisotropic DW chirality inα–φspace. (a) Two-dimensional histogram of experimental DW magnetization data inα−φspace derived from four SPLEEM compound images includingFig. 2b. Colour bar corresponds to the number of pixels on DW centrelines with a givenφandα. Green dashed lines correspond to the histograms inFig. 2e–h. (b) Sketch of DW configurations with respect to DW orientation, inα−φspace: each circle contains a black and a white domain, blue arrows show DW normal vectorsn, red arrows show orientation of in-plane magnetization of the DWs, grey arrows show direction ofKu. Emerald-coloured regions highlight the preferred configurations realized in the Fe/Ni/W(110) system (that is, left-handed DMI andKualong [001]). Left h., left-handed; right h., right-handed. Figure 3: Distribution of anisotropic DW chirality in α – φ space. ( a ) Two-dimensional histogram of experimental DW magnetization data in α − φ space derived from four SPLEEM compound images including Fig. 2b . Colour bar corresponds to the number of pixels on DW centrelines with a given φ and α . Green dashed lines correspond to the histograms in Fig. 2e–h . ( b ) Sketch of DW configurations with respect to DW orientation, in α − φ space: each circle contains a black and a white domain, blue arrows show DW normal vectors n , red arrows show orientation of in-plane magnetization of the DWs, grey arrows show direction of K u . Emerald-coloured regions highlight the preferred configurations realized in the Fe/Ni/W(110) system (that is, left-handed DMI and K u along [001]). Left h., left-handed; right h., right-handed. Full size image To clarify how the system evolves from homochirality for most α / φ combinations to non-chiral Bloch textures at φ =−90° and +90° we quantify the magnetic chirality of mixed DWs by decomposing the magnetization into Bloch- and Néel- components. By plotting the projections of the magnetization unit vector onto the DW tangent- and normal directions the two-dimensional histogram shown in Fig. 3a can be converted into separate histograms of the Bloch and Néel components: for all points on DW centrelines, the projection of the local magnetization unit vector onto the DW tangent, given by sin( α ), contributes to the Bloch-type histogram and the projection onto the DW normal direction, given by cos( α ), contributes to the Néel-type histogram. The resulting histograms are shown in Fig. 4a,b . From these data, we can quantify average chiralities γ B and γ N of the Bloch-type components and Néel-type components by averaging the magnetization projections over all angles α . 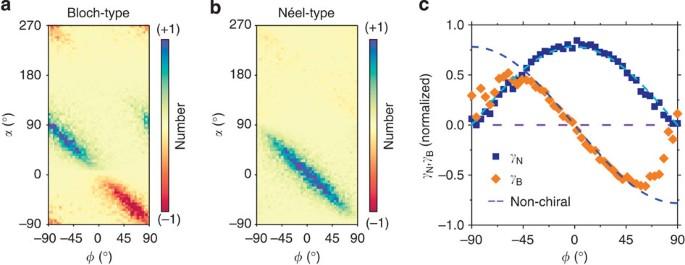Figure 4: Quantifying Néel- and Bloch chirality. Histograms of Bloch wall chirality (a) and Néel wall chirality (b) inα−φspace. (c)φ-dependent chirality of Néel-type (γN) and Bloch-type (γB) components, −1 corresponds to right-handed and +1 corresponds to left-handed. Figure 4: Quantifying Néel- and Bloch chirality. Histograms of Bloch wall chirality ( a ) and Néel wall chirality ( b ) in α − φ space. ( c ) φ -dependent chirality of Néel-type ( γ N ) and Bloch-type ( γ B ) components, −1 corresponds to right-handed and +1 corresponds to left-handed. Full size image The sign of the average chiralities γ B and γ N reflects rotational sense and, following the conventions used by Heide et al . [30] , the Bloch-type component is called left-handed (right-handed) for positive (negative) γ B , and the Néel-type component is left-handed (right-handed) for positive (negative) γ N . Figure 4c plots the dependence of γ B and γ N on φ , the angle between the DW normal and K u . The average Néel chirality is always positive and follows a cosine curve (light blue dashed line), indicating that Néel components of DW spin textures in this system are always left-handed, regardless of the orientation of local DW sections. The average Bloch chirality of DW spin textures follows a sin curve (dark blue dashed line) in the middle region of the plot, where the magnitude of φ is less than ~60°. This indicates that Bloch wall spin texture can be either left-handed or right-handed, depending on the orientation of the DW with respect to the substrate induced anisotropy K u . The sinusoidal φ -dependence suggests that left- and right-handed Bloch components occur with equal likeliness in this system, similar to the case of non-chiral magnets where the DMI can be neglected. Yet this system is clearly different from non-chiral magnets, in which case one would expect the quantities plotted in Fig. 4c to scatter about the flat line where average chirality vanishes, γ =0 (purple dashed line). By contrast, the sinusoidal dependence of average chirality on φ is a result of the anisotropic DMI in the Fe/Ni/W(110) system. Here Bloch chirality gradually vanishes when φ approaches ±90° (ref. 16 ). The gradual deviation from sinusoidal behaviour is interesting because, given that the DMI stabilizes the Bloch-type chirality, measuring how the system evolves from mixed chiral textures at small φ to non-chiral Bloch DWs at φ =±90° offers a way to estimate the strength of the DMI (see Supplementary Note 1 ). A model for the origin of anisotropic chirality Prior work on a similar system, Fe/8 monolayer Ni/W(110), established that in-plane anisotropic strain due to lattice mismatch [31] gives rise to an in-plane uniaxial magnetic anisotropy K u with easy axis along W[001], through magneto-elastic contributions to the magnetic anisotropy [25] . We also confirmed the presence of uniaxial anisotropy K u by SPLEEM observations on thicker in-plane magnetized Fe/Ni films, where the orientation of magnetization of the in-plane domains is always parallel or antiparallel to the W[001] direction. Thus, in these systems, spin structure inside the DWs is a result of interplay between the exchange interaction, the interfacial DMI, the dipolar interaction, the perpendicular magnetic anisotropy, as well as K u . The interfacial DMI favours chiral Néel DWs, and the dipolar interaction favours non-chiral Bloch DWs. Because of its two-fold symmetry, uniaxial anisotropy itself does not influence the chirality of the DWs. However, K u provides an additional force favouring alignment of the magnetization within DWs towards the easy magnetization axis [001]. This additional force lifts the left-/right-handed degeneracy of Bloch-type spin structures whenever DWs are at a non-zero angle with respect to the [001] direction. Simulation for the anisotropic DW To test this model and clarify the role of K u in a DMI system, we performed Monte Carlo simulations [32] , [33] . A two-dimensional Heisenberg model was constructed to simulate DW configurations in the presence of the interfacial DMI and K u (see Supplementary Note 1 ). 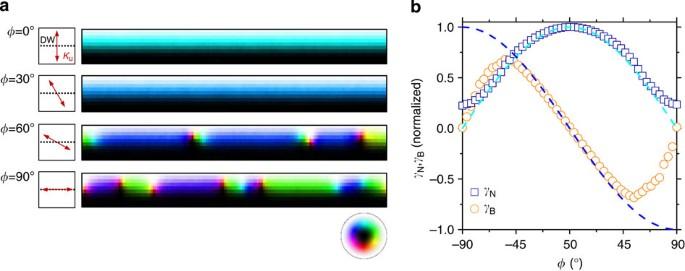Figure 5: Monte Carlo simulation. (a) Monte Carlo simulation results with variable DW orientationφ. White and black regions correspond to perpendicularly magnetized domains, coloured region in between corresponds to DW, and orientation of in-plane component of the DW is highlighted by colour wheel. (b)φ-dependent chiralitiesγNandγBderived from the simulation, −1 corresponds to right-handed and +1 corresponds to left-handed. Figure 5a shows typical simulated DWs. The coloured bars represent straight DW segments, each in a different orientation φ , that is, we sweep the angle φ by changing the easy axis of K u with respect to the DW orientation. As φ varies from 0° to 90°, simulated DWs evolve from chiral Néel-type wall to non-chiral Bloch-type DWs. Quantitative values for the average chiralities γ B and γ N of the Néel- and Bloch- components can be derived from simulation results. Results are shown in Fig. 5b , where the φ dependence of γ B and γ N nicely reproduces the experimental results (see also Supplementary Fig. 2b ). The simulated results suggest that this type of Bloch-component chirality may be a general feature of DMI systems with uniaxial in-plane anisotropy, beyond Fe/Ni/W(110). Figure 5: Monte Carlo simulation. ( a ) Monte Carlo simulation results with variable DW orientation φ . White and black regions correspond to perpendicularly magnetized domains, coloured region in between corresponds to DW, and orientation of in-plane component of the DW is highlighted by colour wheel. ( b ) φ -dependent chiralities γ N and γ B derived from the simulation, −1 corresponds to right-handed and +1 corresponds to left-handed. Full size image Towards a homochiral Bloch-type component In the measurements reported above, both left- and right-handed DW segments coexist within each sample, and the handedness of the chiral Bloch component in DWs in this system is solely determined by the DW orientation φ . This suggests the possibility that the system might be driven into a homochiral state if one can experimentally confine the directions of the DW orientation. One possibility to tune DW orientations might be to fabricate nanowires on W(110). For energetic reasons, DWs in nanowires tend to be oriented orthogonal to the wire direction. By controlling nanowire orientation with respect to the lattice orientation of the tungsten crystal, it may be possible to select preferred DW orientations and thus preferred handedness (and weight) of the Bloch component. Another way to control DW orientations is to exploit the interaction of atomic surface steps with DWs. Results on related thin-film systems have shown how substrate step arrays can be used to orient DWs [34] , [35] . We have confirmed the viability of this approach. Preparing thinner Fe/Ni bilayers, we find that most of the DWs are aligned along surface step directions, as shown in Fig. 6 . Evaluating all DWs in this image shows that the histogram of the angle α has only one peak at −40°, indicating that the Bloch-type chirality in these DWs is right-handed homochiral. Considering that direction and density of atomic surface steps can be controlled by polishing substrates at controlled vicinal angles near the (110) lattice plane, this result suggests that it is indeed possible to prepare Fe/Ni/W(110) structures featuring homochiral DW with tailored Bloch-component spin textures. 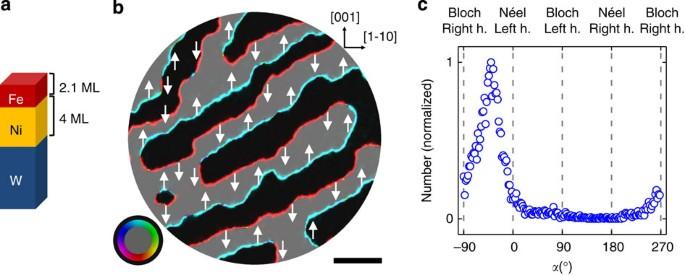Figure 6: Homochiral Bloch-component walls. (a) Sketch of Fe/Ni bilayer grown on W(110) substrate. (b) Compound SPLEEM image highlighting the direction of DW in-plane magnetization. The colour wheel indicates the direction of in-plane magnetization on the DWs. White arrows additionally show the in-plane spin orientations in the DWs; scale bar, 1 μm. (c) Histogram of angleαin DW counted pixel-by-pixel in (b) shows a single peak pointing at ~−40°. Left h., left-handed; right h., right-handed. Figure 6: Homochiral Bloch-component walls. ( a ) Sketch of Fe/Ni bilayer grown on W(110) substrate. ( b ) Compound SPLEEM image highlighting the direction of DW in-plane magnetization. The colour wheel indicates the direction of in-plane magnetization on the DWs. White arrows additionally show the in-plane spin orientations in the DWs; scale bar, 1 μm. ( c ) Histogram of angle α in DW counted pixel-by-pixel in ( b ) shows a single peak pointing at ~−40°. Left h., left-handed; right h., right-handed. Full size image Our experimental results on iron/nickel bilayers epitaxially grown on (110) tungsten surfaces demonstrate that anisotropic chiral magnetism can be stabilized by combining the interfacial DMI with in-plane uniaxial anisotropy. Under these conditions, a family of DW spin textures is stabilized: chiral Néel-type DWs, chiral mixed-type DWs composed of Néel- and Bloch components and non-chiral Bloch-type DWs. The handedness of the Bloch-type component is a function of DW orientation with respect to the substrate lattice, which provides unique opportunities to systematically study in detail the transition between chiral DWs and non-chiral DWs to further understand the interplay between the DMI, magnetic anisotropy and the dipolar interaction. These experimental observations demonstrate how the Bloch-type chirality emerges as a new type of DW spin texture when the interfacial DMI is combined with magnetic anisotropy, thus adding a new degree of freedom to tailor a diverse family of chiral spin textures. The results introduce rich possibilities to influence DW dynamics by combining intrinsic phenomena such as spin Hall effects [18] , [19] , [20] , [21] , [36] , [37] , Rashba effects [18] , [36] , [38] , [39] or the DMI [15] , [18] , not only with magnetoelastically induced anisotropy (as we have shown in this work), but also with piezo-induced strain [40] , [41] , nanowire shape-induced anisotropy [42] or external magnetic fields [19] , [20] , [21] , [43] , [44] , which may open up new opportunities to design spin–orbitronics devices. Sample preparation The W(110) substrate was cleaned by flashing at 1,950 °C in 3 × 10 −8 Torr O 2 and final annealing at 1,900 °C under ultrahigh vacuum with base pressure 4 × 10 −11 Torr. Fe and Ni film thickness was calibrated by monitoring low-energy electron microscopy (LEEM) image intensity oscillations associated with atomic layer-by-layer growth. Fe and Ni layers were grown at 300 K by electron beam evaporation, and the sample was annealed to 900 K for several minutes after growth of one monolayer Ni to develop a well-ordered interface [24] , [25] . Image vector field analysis Two LEEM images, I +p ( i , k ) and I −p ( i , k ), are acquired with spin of the illuminating electron beam aligned and antialigned with a chosen polarization axis p . We typically use image integration times of 1 s. The LEEM images are used to calculate a SPLEEM asymmetry A p ( i , k )=( I +p ( i , k )− I −p ( i , k ))/( I +p ( i , k )+ I −p ( i , k )). The asymmetry value A p ( i , k ) at pixel coordinates ( i , k ) within a SPLEEM image is proportional to the projection of the magnetization vector m ( i , k ) of the sample on the chosen polarization axis p , A P ( i , k )~( m ( i , k )· p ). We choose three orthonormal vectors x , y and z to form a cartesian coordinate system with z being normal to the sample surface. From sets of three SPLEEM images shown in Supplementary Fig. 3a–c , each with p set to be parallel to one of the three components of the sample surface coordinates, the direction of magnetization unit vector m can be determined at all pixel coordinates. To obtain low-noise three-dimensional vector fields A ( i , k ) used for this study, we aligned and averaged 40 such images for the component in the out-of-plane direction ( z ) and 100 each for the in-plane directions ( x , y ). To represent these vector images in colour, we mapped the in-plane angle on hue and the out-of-plane component to the brightness of the image ( Supplementary Fig. 3d ). For higher contrast within DWs, the contrast range of the out-of-plane domains was reduced to 50%. The centrelines of the DWs were determined by thresholding at A z ( i , k )=0 and subtracting the thresholded image from its binary dilation. The DW normal vectors were determined by applying Gaussian blur with a width of 2px and then evaluating the two-dimensional gradient on the centreline. To determine the direction of m ( i , k ), we evaluated and normalized m ( i , k )=( A x ( i , k ), A y ( i , k ),0)/( A x ( i , k ) 2 + A y ( i , k ) 2 ) 1/2 so that the blur of the strong signal of the z component overlapping with the DW does not add noise to the data. Determining m ( i , k ) from single-pixel centrelines and from three-, five- and seven-pixel-wide ribbons straddling the DW centrelines, we had found that the histograms, characterizing DW magnetization direction as a function of the angles α and φ come out nearly identical; therefore, we use DW centre line pixels in the analysis. How to cite this article: Chen, G. et al . Unlocking Bloch-type chirality in ultrathin magnets through uniaxial strain. Nat. Commun. 6:6598 doi: 10.1038/ncomms7598 (2015).